Exposing a dynamical signature of the freezing transition through the sound propagation gap The conventional view of freezing holds that nuclei of the crystal phase form in the metastable fluid through purely stochastic thermal density fluctuations. The possibility of a change in the character of the fluctuations as the freezing point is traversed is beyond the scope of this perspective. Here we show that this perspective may be incomplete by examination of the time autocorrelation function of the longitudinal current, computed by molecular dynamics for the hard-sphere fluid around its freezing point. In the spatial window where sound is overdamped, we identify a change in the long-time decay of the correlation function at the known freezing points of monodisperse and moderately polydisperse systems. The fact that these findings agree with previous experimental studies of colloidal systems in which particle are subject to diffusive dynamics, suggests that the dynamical signature we identify with the freezing transition is a consequence of packing effects alone. The freezing of a liquid into a crystalline solid is just one of numerous first-order phase transitions we experience every day. Yet we understand little about the underlying processes that drive, for example, the transformation of an isotropic fluid, when cooled or compressed beyond a particular point, to a faceted crystal. In the absence of introduced seeds or gradients, the prevailing classical view holds that the crystal nucleates stochastically in the under-cooled, or over-compressed melt. The free energy barrier, given by the difference between the free energy gain, from the transfer of particles from the metastable fluid to the thermodynamically stable crystal, and the free energy loss in creating the crystal-fluid interface, is the main factor that determines the nucleation rate [1] . For moderate/strong undercooling, homogeneous nucleation occurs with sufficient frequency to be detectable in the limited times and sample volumes accessible to experimental and computational studies [2] , [3] , [4] , [5] . These have provided in considerable detail the microscopic kinetics beneath the stochastic step offered by the classical theory. Broadly speaking it is found that following a deep quench or compression, the resulting metastable fluid is structurally heterogeneous—possessing compact amorphous structures from which Bragg reflecting crystals evolve. For weaker undercooling, the barrier to nucleation is large relative to the mean thermal energy and consequently the occurrence of a fluctuation large enough to form a stable nucleus may be too infrequent to capture experimentally. Nonetheless, the crystal phase must start its separation from the metastable fluid at some point in time, no matter how weak the undercooling. However, evidence for distinguishing structural features in weakly under-cooled fluids is tenuous as is the evidence that such features are precursory to the formation of stable crystals [6] , [7] . So, the question is, what changes at the freezing point? An alternative approach to address this question is suggested by more recent work, mainly on particle suspensions [8] , [9] , [10] , [11] , [12] , where qualitative changes in dynamical rather than structural properties are exposed near the freezing point. Most of the studies, discussed above, have been performed on systems of hard spheres. The notion that without the benefit of attractive forces particles somehow coalesce and assemble into crystals may be somewhat challenging. Nonetheless, as demonstrated by some of the earliest computer simulations of the liquid state, a system of identical hard spheres does indeed have a first-order freezing–melting transition [13] , [14] . Packing fractions of the coexisting fluid and crystal phases, φ f =0.494 and φ m =0.545, have also been established by computer simulation [15] . This is a first-order thermodynamic transition and, as such, its location is determined by the (hard-sphere) interactions among the particles; it is independent of the particles’ motions between encounters, be they ballistic or diffusive. So, one might ask; with regard to the mere fact that particles take up space, what is it that causes a mechanism to emerge, at the packing fraction φ f , that could possibly set up the dynamical conditions for nucleation? The hard-sphere system serves as a valuable reference for the determination of structural and thermodynamic properties [16] , [17] of real fluids and also, by extension of Enskog theory, interpretation of their dynamic spectra [18] , [19] , [20] , [21] . Of course, it is not difficult to appreciate that the dynamical consequences of the (hard-sphere) packing constraints are most clearly exposed under conditions where sound is damped. For colloidal systems this damping is effectively accomplished by the suspending liquid [22] , [23] , and isolation of the direct effects of packing constraints is relatively straightforward [10] , [11] , [12] . When particles are subject to Newtonian dynamics, the barest structural dynamics we seek to isolate are coupled to and, consequently, obfuscated by, propagating sound. According to linearized hydrodynamics, the dynamic structure factor comprises the central Rayleigh peak, due to diffusion of heat, and the doublet of Brillouin peaks shifted by the frequency of the acoustic modes [17] , [24] . In addition, we know from dynamic spectra obtained from neutron scattering [18] , [19] , [20] , [21] , [25] and molecular dynamics (MD) computer simulation [26] , [27] , [28] , [29] , when analysed by extensions of hydrodynamic theory, that acoustic excitations extend to wavelengths comparable to the interatomic spacing. These shorter wavelength sound modes are dispersive and are a feature of dense fluids and liquids rather than gases. And on the face of it they would complicate our task of isolating the dynamical effects of packing constraints on the most relevant length scale. It is significant therefore that for some state points, of several simple fluids studied so far, the sound dispersion curves have gaps—spatial windows where sound is overdamped—for wavevectors around the location of the main maximum in the static structure factor [26] , [27] , [28] , [29] . There is, however, no unique model by which linear hydrodynamics may be extended to finite wavevectors [30] , [31] , and the results are prone to appreciable fitting errors. For the hard-sphere system in particular, available results are scanty [26] , [27] . In addition, neither the frequency nor the other parameters that characterize the viscoelastic dynamics is sufficient to expose possible subtle changes in the character of density fluctuations around the freezing point. For these reasons, we introduce an alternative but simpler analysis of the data. In this paper we investigate the time correlation function, C ( q, τ )=< j *( q , 0) j ( q , τ )>, of the longitudinal particle current, j ( q , t ), computed by MD for the hard-sphere fluid as detailed under Methods. In the Results section, we determine that sound becomes overdamped for wavevectors around the position of the main maximum of the structure factor when the volume fraction exceeds 0.45. This is then where the long-time decay of the current autocorrelation function (CAF), is determined entirely by packing constraints among the spheres. We find that the CAF develops an inflection at a volume fraction that coincides with the known freezing point. Accordingly, we identify the emergence of this anomaly as a signature of freezing. In the Discussion section, we consider these results along with a previous calculation of time correlation function of the particle’s velocity and infer that this dynamical signature indicates the onset of quenched in disorder (QID). In conclusion we conjecture on the evolution of the QID towards crystal nuclei. Determination of the overdamping of sound We begin with the one-component hard-sphere fluid. 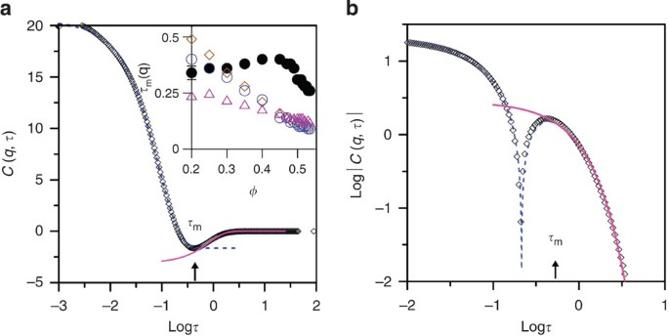Figure 1: Autocorrelation function of the particle current. (a) Linear and (b) logarithmic representations for the packing fraction,φ=0.40, and wavevector,qmd=6.69. The magenta solid line is the fit of the generalised exponential (equation (1)) toC(q,τ>τm). The blue dashed line is a fit of the same function toC(q,τ<τm), drawn here to help delineate fast (τ<τm) from slow (τ>τm) components. The inset inaplots the delay timesτm(q) against packing fraction for wavevectorsqd=2 (brown diamonds),qd=4 (blue circles),qmd(filled black circles) andqd=9 (magenta triangles). Figure 1 shows C ( q , τ ) for the packing fraction φ =0.40, not far below the freezing value, and wavevector, q m d =6.69, where S ( q ) has its main peak. The minimum at the delay time, τ m , delineates what we refer to here as fast ( τ < τ m ) and slow ( τ > τ m ) processes. Qualitatively speaking, C ( q , τ<τ m ) is dominated by the effects of collisions, whereas C ( q , τ>τ m ) is dominated by structural relaxation. Note also from the inset in Fig. 1a that τ m ( q ) shows a broad maximum, around φ =0.45, for the wavevector q m d but it decreases monotonically for the other wavevectors shown. This is already one hint that dynamics exposed around q m d is qualitatively different from that at other values of qd . Figure 1: Autocorrelation function of the particle current. ( a ) Linear and ( b ) logarithmic representations for the packing fraction, φ =0.40, and wavevector, q m d =6.69. The magenta solid line is the fit of the generalised exponential (equation (1)) to C ( q , τ > τ m ). The blue dashed line is a fit of the same function to C (q, τ < τ m ), drawn here to help delineate fast ( τ < τ m ) from slow ( τ > τ m ) components. The inset in a plots the delay times τ m (q) against packing fraction for wavevectors qd =2 (brown diamonds), qd =4 (blue circles), q m d (filled black circles) and qd =9 (magenta triangles). Full size image In what follows, we confine analysis and discussion to the slow process, C ( q , τ>τ m ). Although not shown here, for smaller wavevectors (say qd ≈<1), C ( q , τ>τ m ) exhibits the usual oscillations indicative of underdamped acoustic modes [32] , [33] . However, as we demonstrate below, monotonicity of C ( q , τ>τ m ) at larger wavevectors, as seen in Fig. 1 , for example, like the absence of distinct Brillouin peaks in dynamic spectra [26] , is in itself not sufficient to indicate that sound is overdamped. Our analysis of these data is based on the following reasoning; as C ( q , τ > τ m ) ( Fig. 1a ) is negative, it exposes reversals of the particles’ movements. When such reversals are uncorrelated (in time), as is the case for a dilute system of Brownian particles, the slow fluctuations in the longitudinal current constitute a random Markov process and their time correlation function, C ( q , τ>τ m ), decays by an exponential function of the delay time. Compounding this process by memory of the particles’ momenta mitigates the reversals and advances, or compresses, the decay of C ( q , τ>τ m ) with respect to that of an exponential function. Packing constraints, on the other hand, by the imposition of momentary structural traps cause the decay to be retarded, or stretched, relative to that of the putative Markov process. The Kohlrausch function or generalised exponential (GE) [34] is perhaps the simplest model that encapsulates this gamut of processes [35] . The physically significant parameter here is the exponent γ ( q ) for it distinguishes compression ( γ ( q )>1) from stretching ( γ ( q )<1) of the correlation function. As illustrated in Fig. 1 , we proceed by fitting the GE to C ( q , τ > τ m ). (For completeness, the fit of equation (1) to C ( q , τ < τ m ) is also shown but not considered further in this paper.) The amplitude, K ( q ), time scale, τ x ( q ), exponent, γ ( q ), and the static structure factor are plotted for various packing fractions in Fig. 2 . For reasons discussed below, this part of the analysis is confined to volume fractions φ < φ f . Note that the relaxation rate, , and the amplitude, K ( q ), show minima—particle currents are weaker and slower—for wavevectors around the position, q m , of the main peak in S ( q ), as expected on the basis of de Gennes slowing [36] . For φ <0.45, of which the first panel of Fig. 2 is illustrative, the index, γ (q), exceeds unity for all qd and shows no apparent correlation with S ( q ); whereas, for φ ≈0.45, a hint of such correlation starts to emerge around q m d (≈7), γ ( q ) just starts to reach one. For φ =0.49 Fig. 2 shows that γ goes well below 1 in a range of wavevectors around q m . We have here the situation where, when integrated over the time interval 0 to τ m , the advance of the particle current, due to persistence of the particles’ momenta, is effectively countered by the retard due to the packing constraints: a spatial window emerges where sound is overdamped. So, for φ ≈0.45, q = q m and τ > τ m , the CAF and (by equation (5) under Methods) the intermediate scattering function decays exponentially with delay time. For these conditions, the system of Newtonian hard spheres is statistically equivalent to a system of Brownian particles. 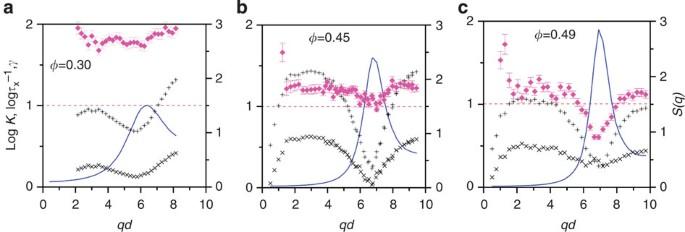Figure 2: Parameters of the generalized exponential of the slow processC(q,τ>τm). Exponent γ, magenta diamonds; amplitude logK, black plusses; relaxation rate, black crosses; structure factor, blue line (right axis). Packing fractions are (a) 0.30, (b) 0.45 and (c) 0.49. The minimum values of these parameters, atq≈qm, are plotted inFig. 4. Figure 2: Parameters of the generalized exponential of the slow process C ( q , τ > τ m ). Exponent γ, magenta diamonds; amplitude log K , black plusses; relaxation rate , black crosses; structure factor, blue line (right axis). Packing fractions are ( a ) 0.30, ( b ) 0.45 and ( c ) 0.49. The minimum values of these parameters, at q ≈ q m , are plotted in Fig. 4 . Full size image In Fig. 3 , we show the sound dispersion curves, obtained by analysis of the MD data by extended hydrodynamics, for packing fractions around the freezing value. One sees that for packing fractions between ~0.45 and 0.50 and a range of wavevectors around qd = q m d ≈7 ω s ( q )=0; that is, there is a propagation gap. Such propagation gaps have been found for other simple fluids around their respective structure factor maxima [19] , [25] , [27] , [29] . Significantly, insofar as the determination of the conditions where sound is overdamped, the results of our procedure based on fitting the GE to the long-time tail of the CAF are consistent with the more conventional analysis. So for these conditions, elastic restoring forces are completely dominated by dissipation. 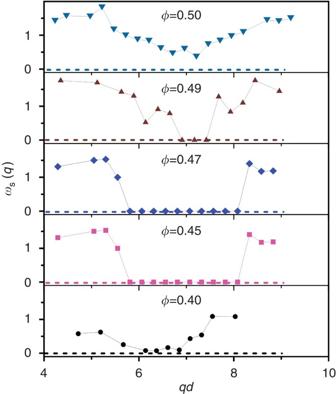Figure 3: Sound dispersion curves. The sound frequency,ωs(q), versus wavevector,qd, for volume fractions indicated. The dashed horizontal lines are drawn to help visualize the gap, which is absent both atφ=0.40 andφ=0.50. Figure 3: Sound dispersion curves. The sound frequency, ω s ( q ), versus wavevector, qd , for volume fractions indicated. The dashed horizontal lines are drawn to help visualize the gap, which is absent both at φ =0.40 and φ =0.50. Full size image Of course the collision frequency among the particles increases with packing fraction. So once, for a given φ (≈0.45), C ( q , τ>τ m ) displays no memory of the collisions ( γ ( q )=1), any further decrease in γ ( q ) or, as we will see below, any deviation of C ( q , τ>τ m ) from the GE, found on increasing φ can be due only to the changes in structural dynamics associated with packing effects alone. Specifically, we suggest that the accompanying increase in heterogeneity of structural traps results in a spread, proportional to γ ( q ) (ref. 35 ), of the currents’ reversal times. The delay time τ x , given by C ( q , τ x )= K ( q )/e, is a measure of the fastest of those times. Values of the parameters, and γ ( q m ) of the SE for the wavevector q m are shown in Fig. 4 as a function of packing fraction. One sees that the value, γ ( q m ), of the exponent decreases further as φ approaches the freezing value. But note also where, for φ ≈0.45, γ ( q m ) drops through unity, the (average) reversal rate, , starts to increase. So, whatever the nature of the collective processes exposed, once sound is overdamped, they become increasingly heterogeneous and dominated by increasingly faster reversals of the particle flux. 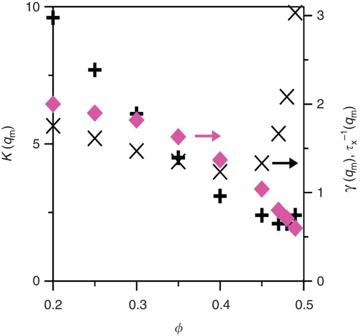Figure 4: Parameters of the generalised exponential atqm. K(qm), black plusses (left axis);, black crosses (right axis);γ(qm) magenta diamonds (right axis). Figure 4: Parameters of the generalised exponential at q m . K ( q m ), black plusses (left axis); , black crosses (right axis); γ ( q m ) magenta diamonds (right axis). Full size image Identification of a dynamical signature of freezing From now on, we restrict our analysis and discussion to the conditions where sound is overdamped, that is, φ >0.45 and q = q m . In the first row of Fig. 5 , log| C ( q m , τ )| is shown for several volume fractions bracketing the known freezing point, φ f =0.494. In all cases known to be in the thermodynamically stable phase ( φ < φ f ), C ( q , τ>τ m ) can be described by the GE function of delay time (equation (1)) within the noise of the data. This is not so for the metastable fluids ( φ > φ f ). Variations in concavity in the decay of the CAF, clearly evident for φ =0.52 ( Fig. 5a ) and φ =0.51 ( Fig. 5b ), suggests the existence of a process, or processes, that distinguish the metastable from the stable fluid. Closer to the transition ( φ =0.50 ( Fig. 5c )), the CAF cannot be described by a GE function nor is there an obvious inflection. Here, over a limited but identifiable time window, |log C ( q , τ )| versus log τ shows no curvature. At this stage, we attach no significance to this lack of curvature in the double logarithm presentation (or apparent power-law decay of C ( q , τ )) other than the means to estimate the packing fraction, φ c =0.500±0.005, where another structural mechanism, specific to the metastable fluid, sets in. There is clearly no suggestion of a discontinuity, at least not to first order in φ . Accordingly, with due regard to noise and resolution of these data, we estimate the packing fraction of the dynamical crossover from the thermodynamically stable to metastable fluid to be 0.50±0.005. 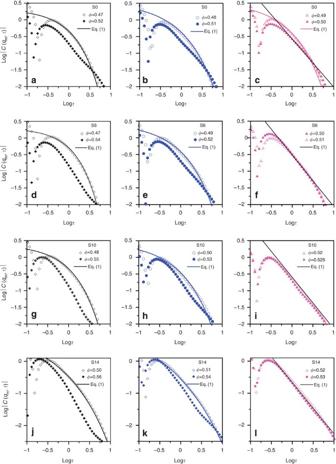Figure 5: Current correlators (CAFs). C(q,τ), for packing fractions,φ, indicated. Only those parts, log|C(q,τ>τm)|, to the right of the respective maxima are relevant to the discussion; the first row, (a–c), are for the one-component hard-sphere fluid, designated S0; the second row, (d–f) are for the system with polydispersity 6%, designated S6; the third row (g–i) are for the system with polydispersity 10%, designated S10; the fourth row (j–l) are for the system with polydispersity 14%, designated S14. Straight lines inc,f,iandlare drawn as a guide to locate the dynamical crossover,φc. Values of the latter obtained from these data, along with estimates of the freezing volume fractions,φf, are listed inTable 1. Figure 5: Current correlators (CAFs). C ( q , τ ), for packing fractions, φ , indicated. Only those parts, log| C ( q , τ > τ m )|, to the right of the respective maxima are relevant to the discussion; the first row, ( a – c ), are for the one-component hard-sphere fluid, designated S0; the second row, ( d – f ) are for the system with polydispersity 6%, designated S6; the third row ( g – i ) are for the system with polydispersity 10%, designated S10; the fourth row ( j – l ) are for the system with polydispersity 14%, designated S14. Straight lines in c , f , i and l are drawn as a guide to locate the dynamical crossover, φ c . Values of the latter obtained from these data, along with estimates of the freezing volume fractions, φ f , are listed in Table 1 . Full size image Results for the polydisperse fluids S6, S10 and S14 are shown in the second, third and fourth rows of Fig. 5 . In Fig. 5d,e for S6, Fig. 5g,h for S10 and Fig. 5j and Fig. 5k for S14, two types of decay in the CAF, one following a SE and the other having some variation in concavity, are evident. This distinction has all but disappeared for example for S6 in Fig. 5f , where, as discussed above for the one-component system, the lack of curvature presents the best way to estimate the packing fraction, φ c =0.505±0.005 in this case, where the dynamical crossover is located. Applying the same criterion to the results for S10 in Fig. 5i and for S14 in Fig. 5l , gives the values of the respective estimates for φ c listed in Table 1 . Table 1 Location of the dynamical crossover. Full size table Estimates of the packing fractions, φ f , of the respective thermodynamic freezing points are also listed in Table 1 . For polydisperse systems [37] , [38] , [39] , these estimates are sensitive to the particle size distribution and, more significantly, whether the protocols allow for fractionation into multiple crystal phases from different sub-populations of the particle size distribution. Then, according to the latest studies [37] , [38] , there is no terminal polydispersity beyond which such phase separation is supressed. However, when fractionation is not taken into account (see ref. 39 and references cited therein), a limiting polydispersity (~10%) is predicted. Clearly, our results for φ c are compatible with those estimates of φ f , based on protocols that allow fractionation. Comparison with experiment Finally, the magnitude of the variation(s) in concavity, increasingly apparent as one goes deeper into the metastable fluid, can be quantified by the (logarithmic) derivative, shown in Fig. 6a . Taking this additional step in processing of the data necessarily incurs some loss of sensitivity to the subtle changes seen in the panels on the right in Fig. 5 . The reason for doing so is that it allows a convenient comparison ( Fig. 6b ) with the corresponding results obtained by dynamic light scattering on a suspension of hard-sphere-like particles [11] . It is clear that for all φ ≤0.49, L ( q m , τ ) decays monotonically for delay time log τ >−0.5 that spans the slow decay of the current correlator. The shoulder in L ( q m , τ ) seen for φ =0.50, around log τ =0, manifests the lack of curvature of C ( q m , τ ) in Fig. 5c . In the metastable phase, at least for φ ≥0.51, the inflections seen in Fig. 5a,b are now manifested by oscillations. In the experimental result ( Fig. 6b ), one sees that non-monotonicity in L ( q m , τ ) sets in when the freezing volume fraction is exceeded. 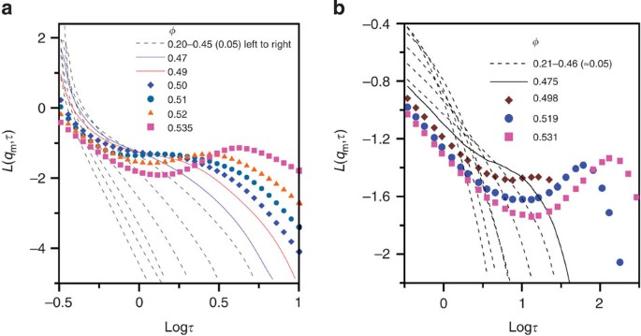Figure 6: Logarithmic derivative of the CAF. L(qm,τ), defined by equation (2) for volume fractions indicated derived from (a) MD for the monodisperse system and (b) experiment, (ref.11). Note the different scales of abscissae and ordinates. While the particles of the experimental samples have a polydispersity of 0.08, the location of the observed first-order freezing transition is referenced to known value of the one-component hard-sphere system49. Figure 6: Logarithmic derivative of the CAF. L ( q m , τ ), defined by equation (2) for volume fractions indicated derived from ( a ) MD for the monodisperse system and ( b ) experiment, (ref. 11 ). Note the different scales of abscissae and ordinates. While the particles of the experimental samples have a polydispersity of 0.08, the location of the observed first-order freezing transition is referenced to known value of the one-component hard-sphere system [49] . Full size image By fitting the GE function of the delay time (equation (1)) to the long-time negative tail of the time autocorrelation function of the longitudinal particle current ( Fig. 1 ), we determine that sound becomes overdamped for wavelengths corresponding to the interparticle spacing for packing fractions of the hard-sphere fluid above φ ≈0.45. In this respect, the results of this novel analysis are consistent with those obtained by the application of extended hydrodynamics. The most significant result of our computations, seen in Fig. 5 , is that the negative ‘tail’, C ( q , τ>τ m ), of the CAF develops a change in concavity or, correspondingly in Fig. 6 , its logarithmic time derivative a maximum. Since this dynamical feature emerges at the freezing volume fraction, φ f , or as near to it as can be determined from the resolution and accuracy of the computations, we propose it to be a dynamical signature of the first-order freezing transition. The consistency, seen in Fig. 6 , of the results of the MD simulations and those of dynamic light scattering experiments on the colloidal system of (diffusing) hard spheres lends further support to the conclusion that, whatever their nature, the ‘modes’ that set in at the freezing point are associated with packing constraints alone; unrelaxed momentum currents in the hard-sphere fluid, or hydrodynamic interactions among the particles sourced from such currents in suspending liquid, have no role, at least not in the time windows of the simulations and experiments discussed here. In addition, Fig. 5 and Table 1 show that as polydispersity is introduced this dynamical signature is relocated in a manner consistent with the predicted relocation of the first-order thermodynamic transition. Extended hydrodynamic analyses also find, by the disappearance of the propagation gap, emergence of another mode at φ ≈0.50. So also, the gap disappears for the fluids with continuous pair potentials at state points rather close to their respective freezing points [28] , [40] . Although fitting errors are appreciable in these analyses, it would be a curious coincidence, nonetheless, if the vanishing of these gaps did not point to the same dynamical signature of freezing as that inferred from our consideration of the CAF. The implication of the connection is that the vanishing of the propagation gap does not signal the re-emergence of sound. To shed some light on the nature of the structural change that occurs or modes that emerge at the freezing point, we consider results of previous studies of the velocity autocorrelation function (VAF), also obtained by MD for the hard-sphere system [8] ; The VAF in the metastable fluid is found to decay by a negative power-law (~− τ −5/2 ) of the delay time [8] . This is fundamentally different from the classical, (positive) hydrodynamic power-law (~ τ −3/2 ) which, in turn, results from the diffusive dissipation of that part of an atom’s instantaneous thermal momentum that is not carried away by sound [41] . A negative power-law is expected in the presence of QID as in the classical Lorentz gas [42] or a porous medium [43] . However, the metastable fluid still flows and, therefore, it does not possess the type of global structural rigidity of a porous solid for example. Presuming that the features of the VAF and the CAF, found in the metastable fluid, have the same origin, we propose that on entering the metastable phase the QID sets in for the wavevector q m . Insofar as it is confined to one wavevector, or as experiments show [10] , [11] , [12] more generally for weakly over-compressed systems, a narrow spread of wavevectors around q m , the QID identified here is too limited, or perhaps too subtle, to quantify the corresponding structural or dynamical heterogeneity (in direct space). At the same time, the emergence of a new source of spatial correlation around q m is not inconsistent with the emergence of amorphous compact structures of which the icosahedron, for example, is one that is manifested by the splitting of the second peak of the radial distribution function [7] , [44] . The latter structural feature is generally adopted to distinguish metastable from thermodynamically stable fluids. Given that nucleation and, therefore, any possible precursory heterogeneous dynamics in these weakly over-compressed fluids are too rare to be observed in typical computer simulations, discussion on the evolution of the QID towards the crystal is necessarily speculative. Our interpretation involves extrapolating our observations to studies, reported elsewhere, of the structure and its evolution in more strongly over-compressed metastable fluids [2] , [3] , [4] , [5] , [6] , [7] . Now, it is evident from Fig. 6 that the oscillation of L ( q m , τ )—a signature of the QID—increases as the degree of over-packing increases. As mentioned already, such enhancement of spatial correlation around q m would be manifested by a sharpening of the main peak, S ( q m ), of the structure factor. Such sharpening is also observed in experimental and computer simulation studies of crystallization kinetics [3] , [4] , [5] of moderately over-packed hard-sphere systems. These find that in the wake of a density quench, but long before Bragg reflections are evident, there is a slow increase of S ( q ) around q m . In turn, this is attributed to the presence of compact amorphous structures. Significantly, it is from these structures that crystal nuclei evolve [3] , [4] , [5] . Accordingly, we can at least speculate that the QID identified here from the combination of previous [8] and current MD simulations is a potential dynamical conduit to nucleation. An obvious alternative possibility is that the QID dissipates after some time, beyond the observation time of the experiments and computer simulations discussed so far. After that, nucleation could then proceed from a dynamically homogeneous fluid by thermal stochastic processes. In this case, our observations of a change in dynamics at the thermodynamic freezing point is no more than an interesting coincidence. Clearly, more extensive experiments and/or computer simulations are required to determine which of these scenarios unfolds in weakly over-compressed fluids. Simulation details Using methods that are now well established [45] , [46] , [47] , we perform event-driven MD simulations in the micro-canonical (NVE) ensemble, after preparation in the canonical (NVT) ensemble, for N =2,000 hard-sphere particles in a cubic box with periodic boundary conditions. For all state points presented in this work, nucleation is too rare/slow to be observed in any practical computational time. Thus, the time correlation functions presented here are invariant to time translation. Particle mass, diameter and mean thermal energy are m , d and k B T (k B is the Boltzmann constant and T the temperature). Length and time are expressed in units of d and d( m /k B T ) 1/2 , respectively. Simulations were carried out for the one-component fluid and for fluids having a spread of particle radii or polydispersity, σ , (width of the distribution relative to the mean) of 0.06, 0.10 and 0.14; respectively designated as S0, S6, S10 and S14. The distribution is given by a 31-component discrete distribution with Gaussian shape [47] . From the trajectories generated, we calculate the intermediate scattering function (ISF), or time correlation function of the particle number density, Here r j ( t ) is the position of the j th particle at time t , q is the scattering vector, τ is the delay time, the asterisk indicates the complex conjugate and the angular brackets indicate the ensemble average of a system of N particles. The ISF has been normalized by the static structure factor, S ( q )=<| ρ ( q )| 2 >. To achieve the statistical accuracy required for the analyses, the reported results are based on at least 600 independent runs, each of duration of up to 10 τ α . Here τ α , defined by f ( q m , τ α )=1/e, is the structural relaxation time of the fluid at the wavevector, q m , where S ( q ) has its main maximum. Calculation of the longitudinal current correlation function The autocorrelation function [17] , [24] of the (longitudinal) particle current (CAF) is obtained by taking the second derivative of the ISF, numerically, with respect to the delay time, Explicitly, the CAF is, where v i ( t ) is the velocity of the i th particle at time t . In the second expression of the CAF both r i ( t ) and v i ( t ) are subject to numerical noise. Since the ISF depends on particle positions only the more efficient avenue, with regard to noise suppression, is to calculate the CAF by equation (5). In Fig. 7 we show that this is indeed the case by comparing the results of direct calculations, via equation (6), with that obtained by equation (5). It is seen that, as the number of independent configurations used in the direct calculation is increased from 14 to 500 to 3,500, the results converge towards those resulting from the second derivative. However, even with the largest ensemble of configurations, the inflection occurring in this case for τ ~2, is only just apparent, whereas the second derivative offers a much better estimate of the inflection with only 500 independent configurations. These results are also in agreement with previous work [48] that found these types of correlation functions can be obtained far more efficiently, without introducing artefacts, by numerical differentiation of correlators dependent on particle positions only. 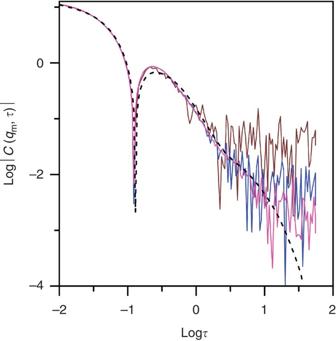Figure 7: Comparison of different routes to calculation of CAFs. |C(q,τ)|, obtained by the second derivative of the ISF (equation (5)) (dashed black line) and calculated explicitly from the particle positions and velocities (equation (6)) (coloured lines) for 14 (brown), 500 (blue) and 3,500 (magenta) independent configurations. Figure 7: Comparison of different routes to calculation of CAFs. | C ( q , τ )|, obtained by the second derivative of the ISF (equation (5)) (dashed black line) and calculated explicitly from the particle positions and velocities (equation (6)) (coloured lines) for 14 (brown), 500 (blue) and 3,500 (magenta) independent configurations. Full size image Extended hydrodynamic analysis In the extended hydrodynamic theory, the ISF is expressed as [25] , [26] , [27] , [28] where A h and z h ( q ) are the real parameters that characterize the extended heat mode and conjugate pairs, A − = A + *, z − ( q )= z + *( q ), the extended sound modes. We performed fits of the right hand side of equation (7) to the ISF by the method of least squares as described in numerous previous works. The only quantity of interest in the present context is the frequency, How to cite this article: Martinez, V. A. et al. Exposing a dynamical signature of the freezing transition through the sound propagation gap. Nat. Commun. 5:5503 doi: 10.1038/ncomms6503 (2014).